Microcavity controlled coupling of excitonic qubits Controlled non-local energy and coherence transfer enables light harvesting in photosynthesis and non-local logical operations in quantum computing. This process is intuitively pictured by a pair of mechanical oscillators, coupled by a spring, allowing for a reversible exchange of excitation. On a microscopic level, the most relevant mechanism of coherent coupling of distant quantum bits—like trapped ions, superconducting qubits or excitons confined in semiconductor quantum dots—is coupling via the electromagnetic field. Here we demonstrate the controlled coherent coupling of spatially separated quantum dots via the photon mode of a solid state microresonator using the strong exciton–photon coupling regime. This is enabled by two-dimensional spectroscopy of the sample’s coherent response, a sensitive probe of the coherent coupling. The results are quantitatively understood in a rigorous description of the cavity-mediated coupling of the quantum dot excitons. This mechanism can be used, for instance in photonic crystal cavity networks, to enable a long-range, non-local coherent coupling. In quantum information science and cavity quantum electrodynamics, the quantum bus technology aims to provide dissipation-less coupling between distant quantum systems. Within this field, long-range coherent coupling between individual, distant superconducting qubits has recently been demonstrated [1] , so that the construction of quantum logic gates and networks is within the reach of present technology [2] , [3] , [4] . In this context, qubits embedded in a solid state matrix are attractive, as they can fully benefit from the lithographic and materials processing techniques developed in the semiconductor industry to fabricate on-demand photonic layouts, so as to enable long-range coherent coupling within a discrete set of qubits via a photonic intra-cavity bus. Moreover, their ‘niche’ with respect to superconducting qubits is marked out by a simultaneous functionality at relatively high temperatures and at optical frequencies, and they provide an interface to flying qubits such as photons in optical fibres. In recent years, significant progress has been made in the realization of high-quality optical microresonators that enabled pioneering demonstrations of the strong [5] , [6] , [7] , [8] and quantum strong coupling regime [9] , [10] in the solid state. Micropillar cavities ( Fig. 1a ) are a model system for the study of strong coupling in this field. They consist of self-assembled InGaAs quantum dots (QDs)–providing individual exciton states of high oscillator strength, located in the anti-node of the fundamental cavity mode (C). In these structures, a quantum of optical excitation coherently oscillates between the fermionic exciton and bosonic cavity photon state. The resulting eigenstates of mixed exciton and photon character form a Jaynes-Cummings ladder [11] , with increasing number of photons in the cavity mode, showing a Rabi splitting of the rungs proportional to the root of the photon number. 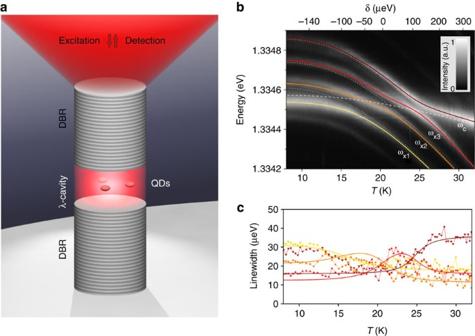Figure 1: Characterization of the investigated quantum dot - micropillar system. (a) Sketch of the micropillar structure including the light coupling from the top facet. (b) Temperature-dependent photoluminescence spectral intensity under non-resonant excitation on a linear grey scale black (0) to white (maximum). The bare resonance energies of excitons and the cavity mode (white dotted lines and dashed line, respectively), and the coupled polariton energies (solid lines) obtained from a Lorentzian lineshape fit and modelling (seeSupplementary Note 2) are overlayed to the data. The corresponding average detuningδ(see equation 1) is shown on the upper axis scale. (c) Coupled resonance linewidths (measured: symbols, modelling: lines). Colours and linestyles as inb. Figure 1: Characterization of the investigated quantum dot - micropillar system. ( a ) Sketch of the micropillar structure including the light coupling from the top facet. ( b ) Temperature-dependent photoluminescence spectral intensity under non-resonant excitation on a linear grey scale black (0) to white (maximum). The bare resonance energies of excitons and the cavity mode (white dotted lines and dashed line, respectively), and the coupled polariton energies (solid lines) obtained from a Lorentzian lineshape fit and modelling (see Supplementary Note 2 ) are overlayed to the data. The corresponding average detuning δ (see equation 1) is shown on the upper axis scale. ( c ) Coupled resonance linewidths (measured: symbols, modelling: lines). Colours and linestyles as in b . Full size image In this article we report on coherent measurements and modelling of cavity-mediated coherent coupling between three QD excitons, moving from the Jaynes-Cummings ladder to the Tavis-Cummings ladder [12] . This constitutes a crucial step towards a quantum bus based on semiconductor photonic structures. Micro-photoluminescence characterization Coherent photonic coupling of distant qubits is realized here by their dipole interaction with a common optical mode of a high-quality microresonator. For this purpose, we have chosen a micropillar similar to that employed in [10] as described in the Methods section. By micro-photoluminescence (μPL) measurements as shown in Fig. 1b , we have identified a triplet of QD excitons—labelled X1, X2 and X3, which at a temperature of 8 K are slightly blue shifted from the cavity mode. Increasing the sample temperature, the excitons (dotted lines) are tuned through the cavity (dashed line) because of the reduction of the semiconductor band gap. The data are consistent with three exciton-cavity avoided crossings at around 13, 21 and 25 K, suggesting that each of the excitonic states is in the strong coupling regime with the cavity mode. A triple exciton-cavity system has a level scheme as shown in Fig. 2 , more complex than the previously studied single-exciton-cavity system [10] . It hosts four polaritonic transitions from the vacuum state. The polariton frequency tuning (solid lines in Fig. 1b ) as well as the variation of polariton linewidths (solid lines in Fig. 1c ) can be described by a coupled oscillator model with the X1-C, X2-C, X3-C coupling parameters eV, homogeneous broadenings eV and frequency distances eV, and eV. The parameters were obtained from a global fit of the coupled oscillator model to the detuning-dependent transition energies and broadenings determined by Lorentzian lineshape fitting of the μPL spectra in Fig. 1b as described in Supplementary Note 2 . 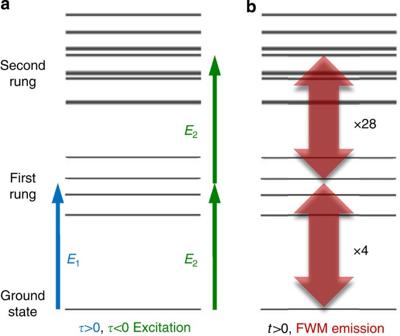Figure 2: Level scheme and relevant transitions. The level scheme of the Tavis-Cummings ladder of the three exciton-one cavity system, and transitions relevant for the coherent FWM response, forδ=−29 μeV. (a) Coherence created by the pulse arriving first (E1for,E2for). (b) Transitions emitting FWM after the arrival of the second pulse. To describe the detuning in this Tavis-Cummings system with non-identical two-level systems, we introduce the average cavity detuning Figure 2: Level scheme and relevant transitions. The level scheme of the Tavis-Cummings ladder of the three exciton-one cavity system, and transitions relevant for the coherent FWM response, for δ =−29 μeV. ( a ) Coherence created by the pulse arriving first ( E 1 for , E 2 for ). ( b ) Transitions emitting FWM after the arrival of the second pulse. Full size image having the values of −124, 16, and 124 μeV at the three anti-crossing points. Multi-polaritonic features as reported in Fig. 1b were previously observed in μPL experiments [13] , [14] and indicate via an anti-crossing behaviour between individual excitons and the cavity mode that excitons could be coherently coupled by the cavity field. However, a direct measurement of coherent coupling is not afforded by μPL measuring the incoherent emission, neither does it provide means to perform coherent optical manipulation in prospective quantum bus nanophotonic structures. An explicit demonstration and selective manipulation of the cavity-mediated coherent coupling of excitons requires extracting and controlling the coherent response of the photonic resonator. Coherent dynamics measured in four-wave mixing To demonstrate and study the cavity-mediated coherent coupling of excitons, we employ here heterodyne spectral interferometry (HSI). [15] This technique—as explained in Supplementary Note 3 —is used to measure the four-wave mixing (FWM) of the strongly coupled exciton-cavity system, which arises from the optical nonlinearity of the QD excitons. In short, two pulses E 1 and E 2 of 1-ps duration and variable delay τ are exciting the fundamental cavity mode, see Supplementary Fig. S5 . The resulting FWM polarization emitted from the micropillar and its Fourier transform versus t , , are measured using spectral interferometry. The coherent dynamics giving rise to FWM involves the four exciton-cavity mixed states of the first rung of the Tavis-Cummings ladder, which were identified in μPL, and additionally the seven polariton states of the second rung which are mixed states of the family of uncoupled exciton–photon states of the second rung: one two-photon state without excitons, three one-photon states with one of the three excitons filled, and three zero-photon states with two of the three exciton states filled. A sketch of the resulting ladder of levels at T =19 K ( eV) is shown in Fig. 2 , together with the transitions relevant for the delay time and real-time coherent dynamics probed in FWM. For positive delay τ >0, pulse E 1 arrives first and creates a one-photon coherence given by a wavepacket of the four states of the first rung, which is coherently evolving until the arrival of E 2 . Conversely, for negative delay τ <0, pulse E 2 arrives first and creates a two-photon coherence given by a wavepacket in the second rung, which is coherently evolving until the arrival of E 1 . In both cases, at the arrival of the second pulse FWM is created as a superposition of all optical transitions between the ground state, first and second rung, consisting of four transitions between the ground state and the first rung and 28 transitions between the first and second rung of the Tavis-Cummings ladder. We calculate the FWM polarization analytically taking into account the states up to the second rung, by solving the master equation for the density matrix using a standard exciton-cavity coupling Hamiltonian and a Lindblad dissipation operator (see Supplementary Note 1 ). This approach is exact for the third-order FWM signal of an initially unexcited system. The resulting measurements and corresponding predictions of FWM of the system are given in Fig. 3 as function of time delay τ for two different detuning parameters. The FWM power for eV ( T= 19 K) is shown spectrally resolved in Fig. 3a and time resolved in Fig. 3c . A dynamics significantly richer than in a single exciton case [10] is observed, as expected from the larger number of levels in the first and second rungs, providing 32 instead of 6 transitions contributing to the FWM (see Fig. 2 ). The time-integrated FWM power and the power at a given time t m =21 ps corresponding to the build-up lag of the FWM in such strongly coupled exciton-cavity systems [10] are presented in Fig. 3e . On a qualitative level, we notice the FWM beat as a function of τ with a period of about 17 ps, corresponding to a spectral splitting of 243 μeV. This is much larger than the Rabi splitting of any individual exciton, indicating that all four polaritons contribute towards the coherent dynamics. In Fig. 3b we present the predicted FWM corresponding to Fig. 3a , using the exciton and cavity parameters retrieved from the μPL data (see Fig. 1 and Supplementary Note 2 ). The prediction, which takes into account the coherent evolution in the Tavis-Cummings ladder shown in Fig. 2 , reproduces the rich features of the measurements quantitatively. 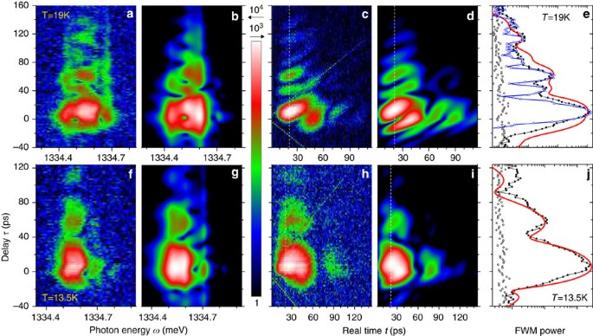Figure 3: Coherent dynamics measured in four-wave mixing. Delay time dependence of the coherent response forT=19 K (top) andT=13.5 K (bottom). Spectrally resolved FWM power, measured (a,f) and predicted (b,g), on a logarithmic colour scale over four orders of magnitude. Time-resolved FWM power, measured (c,h) and predicted (d,i) over three orders. (e,j) Time-integrated FWM power, measured (black circles) and predicted (red line), and measured(blue triangles). The noise ofis given as open circles. Figure 3: Coherent dynamics measured in four-wave mixing. Delay time dependence of the coherent response for T =19 K (top) and T =13.5 K (bottom). Spectrally resolved FWM power , measured ( a , f ) and predicted ( b , g ), on a logarithmic colour scale over four orders of magnitude. Time-resolved FWM power , measured ( c , h ) and predicted ( d , i ) over three orders. ( e , j ) Time-integrated FWM power , measured (black circles) and predicted (red line), and measured (blue triangles). The noise of is given as open circles. Full size image Modifying the detuning, we can adjust the system to exhibit only one exciton in resonance with the cavity, while the other excitons are significantly detuned, so that the dynamics resembles that of a simpler single-exciton-cavity system. This is achieved at eV ( T =13.5 K), for which X1 is in resonance with the cavity within 5 μeV, while X2 and X3 are detuned by 135 μeV and 253 μeV, respectively. The measured and predicted and are presented in Fig. 3f and Fig. 3g , respectively, while the time-integrated FWM is displayed in Fig. 3j . We observe a beat versus delay τ with a period of about 50 ps, corresponding to a polaritonic splitting of 83 μeV, somewhat larger than the calculated splitting of 60 μeV, which is slightly below 2 g 1 due to the finite damping. The faster than expected beat period is due to remaining influence of the two additional excitons, as shown by the agreement of the predicted dynamics including all excitons (see solid line) with the measurements. Cavity-mediated coherent coupling The agreement between the measured FWM dynamics and independently predicted FWM in the framework of the cavity-mediated coupling model for different detunings is revealing the coherent coupling of the three excitons via the cavity mode in the studied microresonator. A definite display of the coherent coupling is afforded by the two-dimensional (2D) frequency domain representation of the FWM, in which coherent coupling is observed as off-diagonal signals [16] , [17] , [18] , [19] . We retrieve the 2D FWM [15] by Fourier-transforming from the delay time τ into the conjugated frequency yielding . In this transformation we use only positive delays , such that represents the frequency of the first-order polarization created by E 1 . The resulting 2D FWM diagram is presented in Fig. 4a . 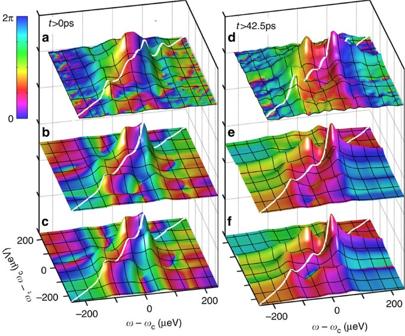Figure 4: Cavity-mediated coherent coupling revealed by two-dimensional FWM. Two-dimensional FWM atT=19 K withmeV.measured and phase corrected (a) and predicted with (b) and without (c) phase correction. The amplitude is given as height, while the phase is given as hue of the surface colour, as indicated. The white line shows the diagonalon the surface. (d–f) As (a–c), but showing the post-selected. Different representations of the data are shown inSupplementary Figs S10 and S11. Figure 4: Cavity-mediated coherent coupling revealed by two-dimensional FWM. Two-dimensional FWM at T =19 K with meV. measured and phase corrected ( a ) and predicted with ( b ) and without ( c ) phase correction. The amplitude is given as height, while the phase is given as hue of the surface colour, as indicated. The white line shows the diagonal on the surface. ( d – f ) As ( a – c ), but showing the post-selected . Different representations of the data are shown in Supplementary Figs S10 and S11 . Full size image To enable the Fourier transformation the relative phase of data at different delays τ needs to be known, but are not measured in the implementation of HSI used here. We therefore employ a phase correction [20] discussed in Supplementary Note 4 , which is estimating this phase. Although this estimation is not exact, and therefore the resulting 2D FWM data deviate from the exact representation, the predictions with and without phase correction given in Fig. 4b and c , respectively, show that this deviation does not qualitatively change the off-diagonal structure. Using the same phase-corrected representation for measurement and prediction they can be quantitatively compared. In the 2D representation, coupled resonances manifest themselves by corresponding off-diagonal components, showing that resonances excited by the first pulse in first order ( axis) coherently couple to a different resonances emitting in third order ( axis). The off-diagonal amplitudes are best visible in the amplitude only representation given in Supplementary Fig. S10 . We note that these off-diagonals are robust in the strong coupling regime, while they gradually disappear when going to the weak exciton–photon coupling, as shown in Supplementary Fig. S14 . Owing to the contributions of the 28 short-lived second-rung transitions, the features in 2D FWM are broadened. Post-selecting the FWM signal emitted after a survival time t s after its creation by the second pulse at t =0, resulting in the 2D FWM , we can suppress the fast decaying components [10] . The measured and predicted post-selected (see Fig. 4d–f ) are therefore dominated by the long-lived first-rung transitions and display a clear separation between the multiple off-diagonals at the polariton frequencies (see Supplementary Notes 1 and 5 ), showing cavity-mediated mutual coherent coupling between excitons. The corresponding data for T =13.5 K ( eV) given in Supplementary Fig. S12 shows the coherent coupling between two polaritonic modes dominated by the cavity and X1. A detailed analysis of the strength of the off-diagonal peaks and their relation to the coherent coupling strength will be presented in a forthcoming work. The observed coherent coupling between three qubits via the cavity mode demonstrates that an optical microcavity can act as a coupling bus for excitonic qubits. The coherent interaction can be controlled by non-local tuning of the cavity mode or the exciton energy, or by switching the excitonic qubit between bright and dark exciton states [21] . Importantly, this coupling mechanism is relevant to all qubit systems that can be controlled by an associated optical transition, such as electron or hole spins in charged QDs [22] , [23] , [24] , and defects in bulk materials such as the NV centre in diamond [25] . The coupling via the cavity mode has the prospect to be spatially extended in coupled cavity structures, for example, in photonic crystals [26] . The small size of the QDs with respect to the cavity enables coupling of many more than three qubits, enhancing the prospects of quantum information processing on a chip with a photonic interface. Samples The fabrication process of high-Q QD micropillar structures starts with the growth of a planar microcavity on an undoped GaAs substrate by molecular beam epitaxy. A GaAs λ -cavity with a single layer of self-assembled In 0.4 Ga 0.6 As QDs with a ground state exciton emission wavelength around 930 nm is sandwiched between two distributed Bragg reflectors (DBRs) providing a vertical photon confinement. The upper (lower) DBR consists of 26 (30) mirror pairs, which are made of λ /4 layers of GaAs and AlAs. For lateral photon confinement micropillars with a nominally circular cross-section and diameters between 1.6 and 2.0 μm were structured by means of high-resolution electron beam lithography and electron cyclotron etching. The fundamental cavity mode in the investigated structure has a Q-factor of 30,000, and a corresponding photon lifetime of about 10 ps within its mode volume of ~0.3 μm 3 . Further details are given in Supplementary Note 2 . FWM experiment We employ HSI [15] , using a pair of pulse trains, E 1 and E 2 , at a repetition rate of 76 MHz and 1-ps pulse duration that are frequency up-shifted by MHz by acousto-optic devices. The spatial mode of E 1 and E 2 is matched to the cavity mode on the top facet of the micropillar by a microscope objective mounted inside a helium bath cryostat. The pulses are resonant to the cavity mode and are injecting into the intra-cavity field in average 0.25 (0.75) photons per pulse of E 1 ( E 2 ), respectively, see Supplementary Fig. S15 . The emitted light is interfered with a frequency unshifted reference field and the FWM signal is selected at the heterodyne beat note and spectrally resolved. The complex FWM response is retrieved by spectral interferometry [15] , [27] . Theory We use a standard approach [13] , [14] , [28] , with the Hamiltonian of a single photonic mode coupled to three two-level systems with dissipation of all components taken into account by a Lindblad super-operator. To calculate the FWM polarization, we follow our earlier rigorous approach [10] , [29] to the optical response of a system on a sequence of optical pulses. For the present system excited by two ultrashort pulses it has the analytic form in which ( ) are the complex polariton frequencies of the first (second) rung, for positive (negative) delay times τ , respectively, while are the complex frequencies of all possible transitions between the ground state and the first rung, and between the first and second rung, all contributing to the real-time dynamics. The expansion coefficients c jk are calculated exactly, reducing the master equation for the full density matrix to a finite matrix problem. Further details are available in Supplementary Note 1 . How to cite this article: Albert, F. et al. Microcavity controlled coupling of excitonic qubits. Nat. Commun. 4:1747 doi: 10.1038/ncomms2764 (2013).